Dissociation dynamics of singly charged vortices into half-quantum vortex pairs The quest for identification and understanding of fractional vorticity is a major subject of research in the quantum fluids domain, ranging from superconductors, superfluid Helium-3 to cold atoms. In a two-dimensional Bose degenerate gas with a spin degree of freedom, the fundamental topological excitations are fractional vortical entities, called half-quantum vortices. Convincing evidence for the existence of half-quantum vortices was recently provided in spinor polariton condensates. The half-quantum vortices can be regarded as the fundamental structural components of singly charged vortices but, so far, no experimental evidence of this relation has been provided. Here we report on the direct and time-resolved observation of the dynamical process of the dissociation of a singly charged vortex into its primary components, a pair of half-quantum vortices. The physical origin of the observed phenomenology is found in a spatially inhomogeneous static potential that couples the two spin components of the condensate. Quantized vortices are topological excitations occurring in a variety of quantum systems, such as Bose–Einstein condensates [1] , [2] , superfluids [3] and superconductors [4] , [5] . Understanding such excitations is therefore fundamental to the study of quantum phases and quantum phase transitions. Semiconductor microcavities in the strong coupling regime proved to be very successful systems for the study of quantum turbulence. The eigenstates of such systems are the so-called exciton-polaritons - bosonic quasiparticles formed in semiconductor microcavities by efficiently coupling the photon cavity mode with a quantum-well exciton resonance [6] . The mixed light-matter nature of such particles confers them favourable properties in view of Bose–Einstein condensation (BEC) at high temperature: the photonic component provides a light mass (10 −4 times the free electron mass) while the excitonic part allows for polariton interactions [7] . The recent experimental demonstration of polariton BEC in many different experimental configurations [7] , [8] , [9] , [10] , [11] , followed by the observation of polariton superfluidity [12] , [13] , has initiated the fascinating field of polariton quantum hydrodynamics. Particular attention has been devoted to the investigation of vortex excitations, both in the case of resonantly driven hydrodynamic experiments [14] , [15] and non-resonant [16] , [17] optical pumping. In the particular case of Bose degenerate gases with spin degree of freedom, commonly known as spinor condensates, the fundamental topological excitations are more exotic vortical entities, called half-quantum vortices (HQVs) [18] , [19] , [20] , [21] , [22] , [23] . They can be conceived as the primary structural components of singly charged vortices (namely vortices with winding number ±1). Being the lowest energy topological excitations, they are essential in determining the Kosterlitz–Thouless phase transition in spinor quantum fluids [22] . Convincing experimental evidence of HQVs was recently provided in a spinor polariton condensate [24] , where the properties of the system allow for direct imaging of both the amplitude and phase of the condensate wave function. Signs of fractional vorticity were previously only reported in high-temperature superconductors [25] , later indirectly measured in spin-triplet superconductors [26] and identified as a result of the decay of 2D Skyrmions in atomic condensates [27] , while their observation is still elusive in other spinor systems like He3 thin films [28] . Spin vortices and textures, which are closely related phenomena to HQVs, have been also investigated in ferromagnetic BEC of 87 Rb atoms [29] , opening the way to an even broader interest in spinor topologies. In this work we investigate the time evolution of a spinor polariton condensate and we report on the real-time dynamics of the unbinding of a full-quantized vortex, appearing at the early instants of the creation of the spinor condensate, into its elementary components: a pair of HQVs. We propose a theoretical model that fully captures the observed phenomenology and provides a well-founded explanation on the origin of the process in terms of a spin-dependent energy landscape. Vortices in spinor polariton condensates Taking advantage of the non-equilibrium condensation mechanism that introduces losses of polaritons by the emission of photons, measurements of the quantum fluid are possible by optical means, as all the properties of the intracavity polariton fluid are inherited by the emitted photons [30] (extracavity field). In particular, the phase and spin of the quantum polariton field are coded, respectively, in the phase and polarization of the emitted light. We therefore make use of both photoluminescence (PL) measurements and advanced time-resolved interferometric techniques to probe the dynamics of the HQV pair generation process from the unbinding of a full quantum vortice (QV). In order to conveniently visualize the vortex unbinding effect, it is worth expressing the linear order parameter of the spinor condensate in the circular polarization basis: where θ ( r ) is the phase, η ( r ) is the polarization angle and n ( r ) is the condensate density. Differently from singly charged vortices (which are characterized by a 2 π phase winding when circumventing the vortex core), the HQVs of spinor condensates involve both a π phase winding and a π polarization rotation, allowed for by the additional spin degree of freedom. In the circular polarization basis, a HQV results in a full 2 π phase shift in one polarization and no phase shift in the other. This feature significantly simplifies the detection method as we make use of a polarization mixing Mach–Zehnder interferometer [24] (see Methods section), in the mirror-retroreflector configuration ( Fig. 1a ). At the input of such an interferometer the two spin components of the same condensate are separated and at its output one polarization is recombined with the retroreflected replica of the other. In this configuration, a singly charged vortex (a vortex occurring in both circular polarization components) manifests as a pair of fork-like dislocations of opposite orientation. This pair appears to be centrosymmetric with respect to the autocorrelation point—the spatial point overlapping with itself—due to the spatial inversion symmetry of the retroreflector ( Fig. 2a ). On the contrary, a HQV (a vortex occurring in only one spin component) appears as a single fork-like dislocation without any centrosymmetric replica ( Fig. 2b ). The substantial difference in the interferometric signature of QVs with respect to HQVs represents a major advantage of the detection scheme employed, making it qualitatively straightforward to identify and distinguish between the two kinds of excitations. Each different topological excitation in our system corresponds to a different interferometric signature, making it possible to univocally identify the kind of vortical entity (see Supplementary Fig. S1 ). 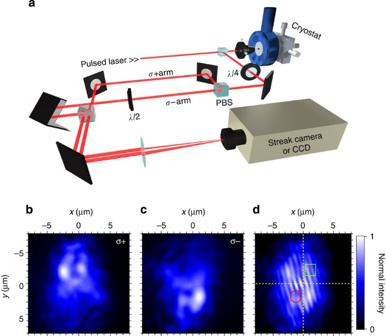Figure 1: Polarization mixing interferometer for vortex detection. (a) Graphical depiction of the experimental setup employed to perform the measurements. The pulsed excitation laser is focused on the sample through a 0.5 numerical aperture (NA) microscope objective, which is also used to collect the PL signal. Using the polarization mixing interferometer we are able to retrieve the mutual coherence betweenσ+(b) andσ− (c) components, thus assessing the spinor nature of the condensate. The presence of QVs or HQVs can be assessed by studying the fork-like dislocations in the interferometric images24(as shown ind). In (d) the yellow dashed lines are a guide to the eye to identify the autocorrelation point. The red circle marks the position of the fork-like dislocation, with straight fringes in the corresponding centrosymmetric position, marked by the green rectangle, thus identifying an half-quantum vortex. Figure 1: Polarization mixing interferometer for vortex detection. ( a ) Graphical depiction of the experimental setup employed to perform the measurements. The pulsed excitation laser is focused on the sample through a 0.5 numerical aperture (NA) microscope objective, which is also used to collect the PL signal. Using the polarization mixing interferometer we are able to retrieve the mutual coherence between σ + ( b ) and σ − ( c ) components, thus assessing the spinor nature of the condensate. The presence of QVs or HQVs can be assessed by studying the fork-like dislocations in the interferometric images [24] (as shown in d ). In ( d ) the yellow dashed lines are a guide to the eye to identify the autocorrelation point. The red circle marks the position of the fork-like dislocation, with straight fringes in the corresponding centrosymmetric position, marked by the green rectangle, thus identifying an half-quantum vortex. 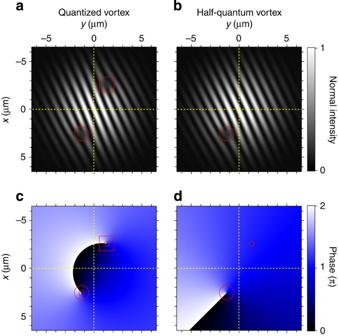Figure 2: Principle of the experiment. The above calculations show the substantial difference between the interferometric signature of a QV and of a HQV when overlapping theσ+with the centrosymmetric replica of theσ−component, in the polarization mixing interferometer. The QV appears as a centrosymmetric pair of fork-like dislocations in the interference pattern (a), corresponding to the phase shown in (c). The red circle and square indicate the phase dislocation positions (large marker) and their corresponding centrosymmetric position (small marker). The HQV instead, appears as only one fork-like dislocation (b) with a 2πphase singularity in the phase structure (d) and no centrosymmetric replica. The yellow dashed lines serve as a guide to the eye and cross each other at the autocorrelation point, central point of symmetry. Full size image Figure 2: Principle of the experiment. The above calculations show the substantial difference between the interferometric signature of a QV and of a HQV when overlapping the σ + with the centrosymmetric replica of the σ − component, in the polarization mixing interferometer. The QV appears as a centrosymmetric pair of fork-like dislocations in the interference pattern ( a ), corresponding to the phase shown in ( c ). The red circle and square indicate the phase dislocation positions (large marker) and their corresponding centrosymmetric position (small marker). The HQV instead, appears as only one fork-like dislocation ( b ) with a 2 π phase singularity in the phase structure ( d ) and no centrosymmetric replica. The yellow dashed lines serve as a guide to the eye and cross each other at the autocorrelation point, central point of symmetry. Full size image Locating the vortices in the sample The sample we use is the CdTe microcavity of our previous work [7] . The non-resonant excitation scheme adopted in the present experiment ensures that no phase structure is imprinted to the condensate and that the phase is indeed spontaneously chosen by the condensation mechanism itself, once the pump power threshold for condensation is crossed. First, we locate specific positions on the surface of the sample where the photonic disorder landscape and the local properties of the sample, in terms of linear polarization splitting [23] , allow for a spinor polariton condensate. The evidence for the spinor nature of such condensates is provided by the presence of HQVs in the time-integrated interferogram acquired with the charge-coupled device (CCD) camera. Overlapping the σ + real-space luminescence pattern ( Fig. 1b ) with the σ − pattern ( Fig. 1c ), we observe clear signatures of HQVs in the interferogram, as marked in Fig. 1d , unveiling the spinor nature of the condensate. Measuring the dynamics of the vortices In order to access the dynamics of the spinor polariton condensate, we image the interferogram, coming from the polarization mixing interferometer, onto the slit of a streak camera. By scanning the position of the imaging lens, we are able to perform a tomographic reconstruction of the real-space interferogram, resolved in time, with ~3 ps time resolution. The experimental results are summarized in Fig. 3 , where the interference patterns (top row) and corresponding phase structures (bottom row) are shown in a set of selected time frames of the dynamics of the spinor condensate. The red circles and squares identify the vortex phase singularities, while the yellow dashed lines intersect at the autocorrelation point. For convenience, we choose the time t =0 to coincide with the instant of arrival of the laser pulse on the sample. In the first frame ( Fig. 3a ) corresponding to the early instants of the condensate creation (35 ps after the pulse arrival on the sample), a full vortex, characterized by a pair of centrosymmetric fork-like dislocations, appears, simultaneously with the long-range coherence of the fluid, close to the centre of the condensate. After a few frames, dissociation of the initially created full vortex into a HQVs pair can be observed, as shown in Fig. 3b . Following this dissociation of the full vortex, one of the created HQVs moves further towards the top edge of the finite-size condensate, while the other HQV remains almost pinned at the initial position ( Fig. 3c ). Eventually, at later times, the two HQVs are pinned by disorder in the spatial positions shown in Fig. 3d , until the end of the condensate decay, thus evidencing the stability of such vortical entities in the spinor system. Quantitative information about the vortex dynamics can be extracted from the data, as shown in Supplementary Fig. S2 . 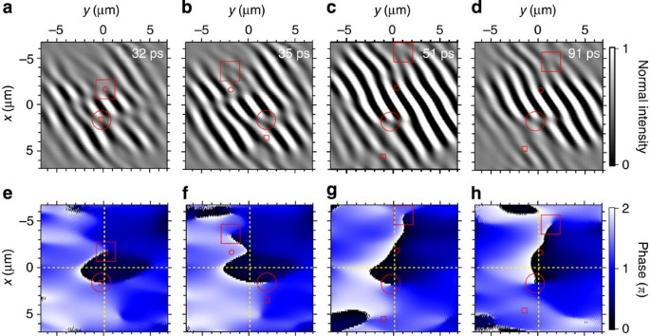Figure 3: Quantized vortex dissociation dynamics. The series of panels summarizes the full vortex unbinding dynamics in the spinor polariton condensate. In the top row we show the interference pattern and the corresponding phase structure (see Methods Section for phase extraction techniques). At the early stages (a,e) a full vortex appears at the centre of the condensate (the red circle and square denote the position of the fork-like dislocations, whereas the small circle and square markers, indicate the respective centrosymmetric position; dashed yellow lines intersect at the autocorrelation point); within a few picoseconds the full vortex dissociates into two HQVs (b,f), corresponding to the two fork-like non-centrosymmetric dislocations (the small markers no longer coincide in space with the respective shapes denoting the singularity position). At later times, one of the HQVs moves towards the top of the condensate while the other remains approximately at the same position (c,g); eventually the HQVs get pinned by disorder in their final positions (d,h). Figure 3: Quantized vortex dissociation dynamics. The series of panels summarizes the full vortex unbinding dynamics in the spinor polariton condensate. In the top row we show the interference pattern and the corresponding phase structure (see Methods Section for phase extraction techniques). At the early stages ( a , e ) a full vortex appears at the centre of the condensate (the red circle and square denote the position of the fork-like dislocations, whereas the small circle and square markers, indicate the respective centrosymmetric position; dashed yellow lines intersect at the autocorrelation point); within a few picoseconds the full vortex dissociates into two HQVs ( b , f ), corresponding to the two fork-like non-centrosymmetric dislocations (the small markers no longer coincide in space with the respective shapes denoting the singularity position). At later times, one of the HQVs moves towards the top of the condensate while the other remains approximately at the same position ( c , g ); eventually the HQVs get pinned by disorder in their final positions ( d , h ). Full size image It is worth noticing that, in the individual time-resolved interference patterns, two fork-like dislocations can be identified, corresponding to the two HQVs. On the contrary, only one fork-like dislocation is clearly visible on the CCD image of Fig. 1d (marked by the red circle). This feature can be understood if one takes into account that the final pinning position of the first HQV (central red circle in Fig. 3d ) is in close proximity to its initial location all along the dynamics and, thus, in a time averaging experiment it leaves a clear signature in the time-integrated CCD image ( Fig. 1d ). On the contrary, the second half-vortex (red square in Fig. 3 ) of the pair travels a long distance and moves during almost all the dynamics, smearing out its trace in the static CCD image, where it cannot be located. Additional information can be extracted by matching the time-resolved and the time-integrated experimental data. The movement of a vortex in time should result in a density minimum path in a time-integrated CCD image, due to the vortex core passing by along its trajectory. Indeed, we found that the trajectories of the HQVs nicely match the density minimum paths in the time-integrated condensate density, each HQV imprinting its trajectory in one of the orthogonal polarization components (see Supplementary Fig. S3 ), confirming that the two HQVs result from the QV dissociation. Theoretical modelling of the dissociation dynamics Theoretically, the physical reason of the QV dissociation is found in a spatially inhomogeneous potential that couples the spin components of the condensate. Such a potential is caused by the weak inhomogeneous energy splitting between the linear polarization components, present in our sample as a result of stress in the microcavity layers. We performed simulations with a model based on the nonlinear driven-dissipative spinor Gross–Pitaevskii equation (GPE), with realistic parameters for the CdTe system (a detailed description and simulation parameters can be found in the Methods section). The results successfully reproducing the QV dissociation effect, are summarized in Fig. 4 . We plot the interference patterns (top row) of four selected time frames of the simulated condensate dynamics and the corresponding phase structure (bottom row). The interferograms of Fig. 4 are obtained by overlapping the σ + and retroreflected σ − component of the condensate, in analogy with the experimental technique. At a certain instant of the condensate dynamics, referred to as t ′=0, two HQVs are seen to enter the condensate following the same spatial path, overlapping to form a full vortex. This is the behaviour of a full-quantized vortex: the QV can be clearly identified ( Fig. 4a ) as the superposition of two HQVs, one in the σ + and the other in the σ − component. After a 5–6 ps, the full vortex is seen to dissociate. Note that this time exceeds the polariton single-particle lifetime and is sufficient to conclude the existence of the QV rather than a simple crossing of the HQV paths. On the other hand, the QV lifetime is short enough to observe the dissociation and the subsequent HQVs dynamics within the effective condensate lifetime. Although the HQV in σ − remains approximately pinned at its initial position ( Fig. 4f ), the HQV in σ + first moves slightly around the former QV position ( Fig. 4b ) to eventually separate in an abrupt way ( Fig. 4d ). 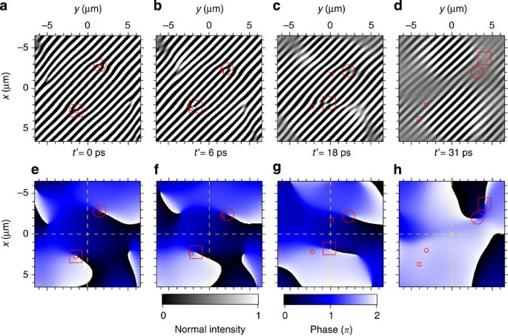Figure 4: Theoretical simulations of quantized vortex dissociation. In these panels we show the QV unbinding dynamics that results from the theoretical simulations. For each time frame, we provide both the interferogram (top row) and the corresponding phase structure (bottom row) of the spinor condensate. Att′=0 ps (a,e) a full vortex appears at the centre of the condensate as a pair of symmetric fork-like dislocations (the position of the HQVs are marked by the red square and circle forσ+andσ−components, respectively, while the corresponding small markers indicate the centrosymmetric position); within a few picoseconds the QV dissociates into two spatially separated HQVs, marked by non centrosymmetric dislocations (b,f). The HQV inσ−remains almost pinned at its initial position (f–h), while the HQV inσ+rapidly moves away (c,d) to eventually abruptly move out of the centre of the condensate (e). Figure 4: Theoretical simulations of quantized vortex dissociation. In these panels we show the QV unbinding dynamics that results from the theoretical simulations. For each time frame, we provide both the interferogram (top row) and the corresponding phase structure (bottom row) of the spinor condensate. At t′ =0 ps ( a , e ) a full vortex appears at the centre of the condensate as a pair of symmetric fork-like dislocations (the position of the HQVs are marked by the red square and circle for σ + and σ − components, respectively, while the corresponding small markers indicate the centrosymmetric position); within a few picoseconds the QV dissociates into two spatially separated HQVs, marked by non centrosymmetric dislocations ( b , f ). The HQV in σ − remains almost pinned at its initial position ( f – h ), while the HQV in σ + rapidly moves away ( c , d ) to eventually abruptly move out of the centre of the condensate ( e ). Full size image We stress the importance of disorder in our sample, which is essential for breaking of the spatial symmetry. First, despite the random initial phase in the fluid and the pulse to pulse variations, the disorder creates preferential paths for vortices such that they appear at similar locations and times in most pulses and can be observed in pulsed averaged experiments. It is then possible, as we report in the present experiment, that some disorder landscapes, upon non-equilibrium condensation of polaritons, make it possible to have the formation of QVs in the first place, which is then followed by the dissociation process into HQVs pair according to the mechanism we described. Any mechanism that does not include spatial symmetry breaking cannot account for vortex observation in pulse averaged experiments with non-resonant (incoherent) excitation, as phase singularity locations would be random from pulse to pulse. The spatial symmetry breaking also fixes the direction of circulation (sign of the vortex winding numbers) as the system is no longer invariant under inversion of the flow directions. Furthermore, to observe half-vortices, the symmetry between σ + and σ − must also be broken. Non-resonant excitation is expected to introduce incoherent excitations with no preferred polarization or phase. In this case, even with a spatially uniform linear polarization splitting, the system would remain invariant under the interchange of σ + and σ − fields. Although it would still be possible to create half-vortices within a given pulse, the initial condensate distribution with σ + and σ − fields interchanged would be equally likely in another pulse. Thus, a half-vortex with the same dynamics but opposite circular polarization would appear with the same probability. Pulse averaging would then give polarization independent results, revealing full vortices at best. A linear polarization splitting with spatially varying direction in the microcavity plane is needed to break the symmetry between σ + and σ − fields. The model we employed in this work shares several elements with the spinor models recently introduced in refs 31 , 32 . In our case, however, as explained, an inhomogeneous birefringence field ( Supplementary Fig. S4 ) has to be simulated to represent the symmetry breaking between σ + and σ − polarizations. An explicit simulation of the reservoir dynamics is also required to model the time dependence of our pulsed experiment [31] , [32] . In this work we have reported on the direct measurement, with picosecond time resolution, of a spontaneous unbinding process of a full vortex into its fundamental components, a pair of HQVs. Our observation unveils one possible generation process of HQVs in polariton condensates and assesses them as dynamical entities. The experimental results are reproduced by means of a spinor generalized GPE, where the novel and fundamental feature is the definition of a disorder dependent static field that couples the spin components of the condensate. The mechanism of QV dissociation discussed in this work sheds light on a dynamical process for HQVs that, with due analogy, could be extended to other spinor quantum fluids. The HQVs are also shown to be capable of long-distance propagation without dephasing. Insight into and control over polariton quantum degrees of freedom opens the perspective of quantum device operation and sets the basis of the new fascinating field of polaritronics [33] . Experimental setup The sample, the same CdTe semiconductor microcavity of ref. 7 [7] , featuring a Rabi splitting of 26 meV, is kept in a cold-finger cryostat at liquid helium temperature (≈4 K). The non-resonant pulsed optical excitation (detuned by ~42 nm with respect to the bottom of the lower polariton branch), provided by a Ti:Sapphire mode locked laser, consists of a train of pulses of ~150 fs at 80.7 MHz repetition rate. The laser is focused onto the surface of the sample with a 0.5 numerical aperture microscope objective. The PL coming from the sample is collected with the same objective and sent to the detection side of the setup. The PL emission of the spinor polariton condensate consists of both σ + and σ − polarization components. The circular polarization components are transformed into cross-linear polarizations using a λ /4 wave-plate and then sent to the polarization mixing interferometer. Its working principle can be summarized as follows: the input polarizing beam-splitter (PBS) separates the cross-linear polarizations (corresponding to the σ + and σ − components of the condensate PL emission). The signal in the so-called σ + arm is left unchanged while the signal in the other interferometer arm, the σ − arm, goes through a λ /2 wave-plate, which is oriented in such a way to make the polarization of the two arms collinear. The σ − arm signal is then retroreflected, thus realizing a centrosymmetric replica of it, and recombined with the σ + beam to get an interference pattern. In the interferogram, as one of the two PL arms is retroreflected, we are able to probe the spatial coherence between points that are far away from each other in the condensate and belong to the two different polarization components. Therefore, the presence of interference fringes is the signature of the long-range mutual coherence between the two polarization (spin) components, confirming that together they compose a spinor condensate and not two independent condensates with orthogonal polarization. Phase extraction technique From the interference pattern in real space we extract the phase structure of the condensate using digital holographic techniques, as implemented in our previous work. In short: the interferogram image is transformed with a 2D FFT algorithm and, because of the applied interference fringes, the oscillatory part carrying the phase information can be isolated in reciprocal space in order to extract the phase information. Finally, a reference phase corresponding to a clean fringe pattern is subtracted to obtain the polariton condensate phase. Theoretical simulation of the condensate dynamics Theoretically, the spatial dynamics of polariton condensates is described by a Gross–Pitaevskii (GP) type equation for the polariton field, coupled to one or more reservoirs that model the dynamics of hot excitons [34] . In reality, not all exciton states in the reservoir contribute to the scattering into the polariton fluid. In order to capture correctly this feature, it is now acknowledged that the GP model must include two coupled reservoirs. An ‘active’ one, from which scattering to the condensate occurs, and an ‘inactive’ one, to account correctly for the reservoir density of states [16] . Excitons in the ‘active’ exciton reservoir, with density n A, σ ( r , t ) fulfil energy momentum conservation laws for scattering into lower polariton states and are described by the rate equation: Here, the polarization components are described by the index σ =±. The parameter R R is the rate of stimulated scattering from the reservoir into the polariton fluid and Γ A is the inverse lifetime of excitons. The active excitons are not directly injected by the pulsed pump, P( r , t ), which rather drives the inactive exciton reservoir, with density n B, σ ( r , t ): Some inactive excitons decay, at rate Γ B , while others are transferred to the active reservoir at a rate τ R This latter process could be mediated by several interactions with phonons, which allow excitons to change their energy and momentum. The pump, which was linearly polarized in our experiment, is assumed to excite the two spin populations equally. Spin relaxation processes in the dynamics of the reservoirs are considered to be negligible on the timescale considered here. For this reason we do not model the presence of dark excitons. We use driven-dissipative GPE to describe the evolution of the polarized polariton fields: where we assumed a parabolic dispersion of polaritons, described by an effective mass m. Interactions between condensed polaritons with parallel and antiparallel spins are described by interaction strengths α 1 and α 2 , respectively. The potential term V 0 represents the disorder in the system, which was modelled by a randomly generated Gauss correlated disorder [35] . The polariton potential is further modified by a blueshift from interaction with the reservoirs, described by strength g R . Polaritons decay from the system at a rate Γ C . In order to model the randomness of the initial conditions of each laser pulse in the experiment, we introduce stochastic initial conditions in the equation. Generation mechanism of half-vortices To generate half-vortices, it is necessary to introduce an asymmetry between the ψ + and ψ − fields. One possible source of asymmetry could be the stochastic element introduced in our model by the initial condition ψ σ ( r , t =0)= θ ( r )/(2Δ r ) where θ is a stochastic white noise with correlator 〈 θ ( r ) θ ( r ′ )〉=2 δ ( r - r ′) and Δ r is the grid spacing. This initial noise is sufficient to seed condensation into the polariton field. equations 2, 3, 4 can be solved numerically for the time dynamics of the system. Physically, a single realization of the noise can be interpreted as modelling the behaviour of an individual pulse in the experiment. To model the experiment, which averages over multiple pulses, we must average over multiple noise realizations. We note that this procedure averages out the asymmetry in polarizations introduced by the noise and the initial noise alone is thus insufficient to describe the appearance of half-vortices in pulse averaged experiments. In order to capture the physics of the HQVs, a further mechanism of induced polarization asymmetry is therefore required. This is to be found in a spatially inhomogeneous static potential, coupling the two spin components of the condensate. In the case of our system, such a potential is provided by the presence of a weak spatially varying energy splitting between linear polarization components. The linear polarization splitting is caused by stress in the sample, which is also the underlying cause of the fluctuating disorder potential. The polarization splitting, coupling between the ψ + and ψ − , and can be modelled by relating its magnitude and direction to the gradient of the disorder potential: where φ is the direction of the vector , that is, tan( φ )= y V 0 / x V 0 , and δE is a constant. We studied a range of different disorder potentials and we found that the spatially varying polarization splitting allows half-vortices to be generated along specific paths that are independent of the initial noise. This allows half-vortices to be observed in experiments averaging over multiple pulses. Simulation parameters The polariton effective mass, was 10 −4 of the free electron mass 16; α 1 =2.4 × 10 −3 meV μm 2 (as in refs 16,36 [16] , [36] ); α 2 =−0.2 α 1 (as in refs 36,37 [36] , [37] ); The polariton decay rate, Γ C =0.2 ps −1 , was matched to experimental measurements of the polariton linewidth; Γ A =15 ps −1 (as in ref. 16 [16] ); Γ B =1 ns −1 (as in ref. 16 [16] ); ħ t R =0.01 meV was chosen to reproduce the effective condensate lifetime ~50 ps as measured experimentally; ħ R R =0.1 meV μm 2 (as in refs 16,34 [16] , [34] ); g R =0.2 × 10 −3 R R was chosen to reproduce the experimentally measured blueshift ~1 meV. The disorder potential was characterized by a correlation length of 2 μm and root mean squared variation 0.2 meV. These parameters are in agreement with previous experimental results studying disorder sensitive effects in our system [7] , [16] . The polarization splitting had a root mean squared value of 2 μev. We considered 500 different realizations of the initial noise. F.M. and K.G.L. performed the experiments and data analysis. T.C.H.L. and V.S. developed theoretical modelling. T.C.H.L. performed the numerical simulations. R.A. grew the sample. B.D. supervised the whole project. All authors contributed to numerous discussions, data analysis and editing of the manuscript. How to cite this article: Manni, F. et al. Dissociation dynamics of singly charged vortices into half-quantum vortex pairs. Nat. Commun . 3:1309 doi: 10.1038/ncomms2310 (2012).